Suppressor of Deltex mediates Pez degradation and modulatesDrosophilamidgut homeostasis Pez functions as an upstream negative regulator of Yorkie (Yki) to regulate intestinal stem cell (ISC) proliferation and is essential for the activity of the Hippo pathway specifically in the Drosophila midgut epithelium. Here we report that Suppressor of Deltex (Su(dx)) acts as a negative regulator of Pez. We show that Su(dx) targets Pez for degradation both in vitro and in vivo . Overexpression of Su(dx) induces proliferation in the fly midgut epithelium, which can be rescued by overexpressed Pez. We also demonstrate that the interaction between Su(dx) and Pez, bridged by WW domains and PY/PPxY motifs, is required for Su(dx)-mediated Pez degradation. Furthermore, we find that Kibra, a binding partner of Pez, stabilizes Pez via WW–PY/PPxY interaction. Moreover, PTPN14, a Pez mammalian homolog, is degraded by overexpressed Su(dx) or Su(dx) homologue WWP1 in mammalian cells. These results reveal a previously unrecognized mechanism of Pez degradation in maintaining the homeostasis of Drosophila midgut. The protein tyrosine phosphatase Pez is the Drosophila homologue of non-receptor type protein tyrosine phosphatase 14 (PTPN14), a regulator of the TGF-β pathway [1] , [2] , [3] . PTPN14 overexpression activates TGF-β signalling and causes epithelial–mesenchymal transition (EMT) [2] . Its overexpression is also correlated with lymphatic function, choanal development, angiogenesis and hereditary haemorrhagic telangiectasia [4] , [5] . Recent studies have revealed that PTPN14 negatively regulates the oncogenic function of Yes-associated protein (YAP) through retaining YAP in the cytoplasm and sustaining the phosphorylation state of YAP [6] , [7] , [8] , [9] . YAP is the transcription co-activator downstream of Hippo signalling to mediate the expression of various genes to promote growth, and its upregulation was found in a variety of human tumours and cancers [10] , [11] , [12] . Drosophila midgut, where the intestinal stem cells (ISCs) are under tight control to maintain homeostasis, has been developed as an excellent model to study adult stem cells in recent years [13] , [14] . The Hippo signalling pathway has been shown to play an essential role in the regulation of ISC proliferation [15] . Pez has been identified as a negative upstream regulator of Yorkie (Yki), the Drosophila homologue of YAP, and is required for the activity of the Hippo pathway in the regulation of ISC proliferation [16] . However, how the stability and function of Pez are regulated remains unclear. Suppressor of Deltex (Su(dx)) is a member of the NEDD4 (neural precursor cell-expressed developmentally downregulated gene 4) family E3 ubiquitin ligase [17] . There are three typical NEDD4 family members in Drosophila , dSmurf, Su(dx) and NEDD4. Each of them contains an N-terminal phospholipid binding C2 domain, four WW domains and a C-terminal HECT-type ligase domain. Su(dx) was first reported as a negative regulator of the Notch signaling pathway [18] . It downregulates the expression of Notch target genes through promoting Notch endosomal sorting [19] , [20] . In this study, we show that Su(dx) targets Pez for degradation both in vitro and in vivo . Su(dx) overexpression induces cell proliferation in Drosophila midgut by downregulating Pez protein levels. We also demonstrate that Su(dx) directly interacts with Pez via its WW domains and Pez’s PY/PPPY motifs. This interaction subsequently promotes Pez ubiquitylation. Furthermore, we find that Kibra, a WW domain containing Pez binding partner, stabilizes Pez on interaction. Moreover, we provide evidence that overexpression of Su(dx) or its homologue WWP1 is able to degrade PTPN14 in mammalian culture cells, indicating a possibility that a conserved mechanism of Pez degradation may play an essential role in maintaining tissue homeostasis. Su(dx) governs Pez stability against proteasomal degradation Drosophila Pez is a newly identified component of the Hippo signalling pathway and specifically functions to restrict the growth of adult midgut epithelium [16] . To date, the degradation mechanism of Pez remains poorly defined. Pez contains multiple proline-rich motifs, which can associate with WW domains to mediate protein–protein interaction [21] . Therefore, we speculated that Pez is likely to be a substrate of WW domain containing NEDD4-like ubiquitin E3 ligases. Screening of NEDD4 family HECT (homologous to E6-associated protein C-terminus) E3 ligases, such as dSmurf, Su(dx) and NEDD4, showed a marked decrease of Pez protein levels when one of the NEDD4 family E3 ligase Su(dx) was coexpressed in S2 cells ( Fig. 1a ). Notably, treatment of proteasome inhibitor MG132 reversed the decrease of Pez protein levels ( Fig. 1b ). The amino-acid Cysteine 917 of Su(dx) is a crucial residue responsible for HECT domain catalytic activity [17] . Coexpression of a Su(dx) mutant protein that contains a cysteine-to-alanine substitution at 917 residue (Su(dx)C917A) failed to promote Pez degradation ( Fig. 1b ). Therefore, Su(dx) regulates Pez protein levels in a proteasome-dependent manner as well as a catalytic activity-dependent manner. Furthermore, coexpression of Su(dx), but not Su(dx)C917A, decreased Pez protein levels in a dosage-dependent manner ( Supplementary Fig. 1a ). To verify if Su(dx) truly induces Pez destabilization, we checked whether the Su(dx) depletion induces changes in endogenous Pez protein levels. A significant stabilization of endogenous Pez was observed on depletion of Su(dx) expression by Su(dx) dsRNA ( Fig. 1c ). The reliability of Pez antibody was confirmed as endogenous Pez was efficiently knocked down by Pez dsRNA in S2 cells ( Supplementary Fig. 1b ). Of note, Su(dx) dsRNA can effectively knockdown Su(dx) at both mRNA level and protein level without impacts on Pez mRNA level ( Supplementary Fig. 1c,d ). In addition, we monitored the level of the transfected Flag-Pez after treatment of the protein synthesis inhibitor, cycloheximide (CHX). We found that knockdown of Su(dx) markedly increased the half-life of Flag-Pez ( Supplementary Fig. 1e,f ). Collectively, Pez stability is regulated by Su(dx) in proteasome-dependent and catalytic activity-dependent manners in S2 cells. 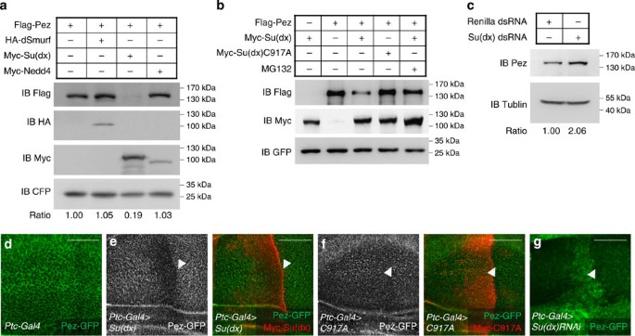Figure 1: Su(dx) promotes Pez degradationin vitroandin vivo. (a) Pez is specifically degraded by Su(dx). S2 cells were transfected with the indicated constructs, and cell lysates were analysed using western blot with the indicated antibodies. CFP was used as a loading control. The quantitative analysis of Flag-Pez/CFP was reported at the bottom. (b) Su(dx) induces proteasome-dependent degradation of Pez. S2 cells were transfected with Flag-Pez and Myc-Su(dx) or Myc-Su(dx)C917A, and treated with or without MG132, followed by western blot analysis. (c) Endogenous Pez protein is stabilized in Su(dx)-knockdown S2 cells. Western blot analysis of endogenous Pez of lysates from S2 cells treated with Renilla dsRNA or Su(dx) dsRNA. Tubulin was used as a loading control. The quantitative analysis of Pez/tubulin was reported at the bottom. (d) Pez distributes evenly inDrosophilawing discs. Immunostaining of the wing discs expressing the GFP-tagged Pez genomic rescue construct (Pez-GFP; stained with GFP antibody, green). Scale bar, 50 μm. (e) Overexpressing Su(dx) causes downregulation of Pez-GFP. Wing discs expressingUAS-Myc-Su(dx)under the control ofPtc-Gal4were immunostained to show Pez-GFP (green) and Myc-Su(dx) (red). White arrowheads indicate the change of Pez-GFP. Scale bar, 50 μm. (f) Overexpressing Su(dx)C917A does not affect Pez-GFP. Wing discs expressingUAS-Myc-Su(dx)-C917Aunder the control ofPtc-Gal4were immunostained to show Pez-GFP (green) and Myc-Su(dx)-C917A (red). Scale bars, 50 μm. (g) Pez-GFP levels are increased when Su(dx) is knocked down. Wing discs expressingUAS-Su(dx)RNAiwithPtc-Gal4were immunostained with GFP (green). White arrowhead indicates the change of Pez-GFP. Scale bar, 50 μm. Figure 1: Su(dx) promotes Pez degradation in vitro and in vivo . ( a ) Pez is specifically degraded by Su(dx). S2 cells were transfected with the indicated constructs, and cell lysates were analysed using western blot with the indicated antibodies. CFP was used as a loading control. The quantitative analysis of Flag-Pez/CFP was reported at the bottom. ( b ) Su(dx) induces proteasome-dependent degradation of Pez. S2 cells were transfected with Flag-Pez and Myc-Su(dx) or Myc-Su(dx)C917A, and treated with or without MG132, followed by western blot analysis. ( c ) Endogenous Pez protein is stabilized in Su(dx)-knockdown S2 cells. Western blot analysis of endogenous Pez of lysates from S2 cells treated with Renilla dsRNA or Su(dx) dsRNA. Tubulin was used as a loading control. The quantitative analysis of Pez/tubulin was reported at the bottom. ( d ) Pez distributes evenly in Drosophila wing discs. Immunostaining of the wing discs expressing the GFP-tagged Pez genomic rescue construct (Pez-GFP; stained with GFP antibody, green). Scale bar, 50 μm. ( e ) Overexpressing Su(dx) causes downregulation of Pez-GFP. Wing discs expressing UAS-Myc-Su(dx) under the control of Ptc-Gal4 were immunostained to show Pez-GFP (green) and Myc-Su(dx) (red). White arrowheads indicate the change of Pez-GFP. Scale bar, 50 μm. ( f ) Overexpressing Su(dx)C917A does not affect Pez-GFP. Wing discs expressing UAS-Myc-Su(dx)-C917A under the control of Ptc-Gal4 were immunostained to show Pez-GFP (green) and Myc-Su(dx)-C917A (red). Scale bars, 50 μm. ( g ) Pez-GFP levels are increased when Su(dx) is knocked down. Wing discs expressing UAS-Su(dx)RNAi with Ptc-Gal4 were immunostained with GFP (green). White arrowhead indicates the change of Pez-GFP. Scale bar, 50 μm. Full size image To determine whether Su(dx) mediates Pez degradation in vivo , we monitored endogenous Pez protein levels in Drosophila imaginal discs. We used a functional GFP-tagged Pez (Pez-GFP), which is encoded by a genomic rescue construct, to indicate the endogenous Pez protein levels ( Fig. 1d ) [16] . Pez RNAi transgene (v40743) was expressed under the control of the patched-Gal4 ( Ptc-Gal4 ) driver, which drives gene expression in a stripe of anterior compartment cells along the anterior/posterior (A/P) compartment boundary of imaginal discs. A stripe of decreased Pez-GFP signal intensity was detected when Pez expression was inhibited (compare Supplementary Fig. 1h with Supplementary Fig. 1g ). As expected, overexpression of Su(dx) under the control of Ptc-Gal4 resulted in a decreased Pez-GFP level in this region (compare Fig. 1e with Fig. 1d ), suggesting that Pez protein levels are downregulated. In contrast, expression of Su(dx)C917A did not affect Pez-GFP levels ( Fig. 1f ), which is consistent with our in vitro data. Moreover, we examined the effects of Su(dx) knockdown on Pez protein levels. As shown in Fig. 1g , knockdown of Su(dx) by Ptc-Gal4>Su(dx)RNAi significantly upregulated Pez-GFP expression in wing discs. Taken together, these observations suggest that Su(dx) regulates Pez protein stability both in vitro and in vivo . Su(dx) overexpression induces intestinal proliferation A previous study reported that Pez functions in Drosophila midgut [16] . We then tested whether Pez is degraded by Su(dx) in midgut. Pez-GFP was evenly expressed in adult midgut ( Fig. 2a , Supplementary Fig. 2a ), and it decreased markedly when Su(dx) was overexpressed in EC cells using a Myo1A ts -Gal4 driver ( Fig. 2b ). In contrast, Pez-GFP levels was not affected in midgut overexpressing Su(dx)C917A ( Fig. 2c ). Moreover, Su(dx) knockdown by RNAi increased Pez-GFP expression ( Fig. 2d ). These results were confirmed by western blot analysis ( Fig. 2e ). On the basis of these findings, we concluded that Su(dx) regulates Pez stability in Drosophila midguts. 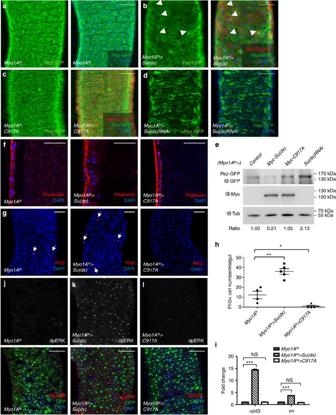Figure 2: Su(dx) overexpression in enterocytes inducesDrosophilaadult gut proliferation. (a) Pez distributes evenly inDrosophilamidgut. Adult fly midguts expressing the GFP-tagged Pez genomic rescue construct (Pez-GFP) were immunostained with GFP (green) and DAPI (blue). Pez distributes evenly inDrosophilamidgut. Scale bar, 50 μm. (b) Overexpressing Su(dx) induces Pez-GFP downregulation. Adult fly midguts expressingUAS-Myc-Su(dx)byMyo1Ats–Gal4were immunostained using Pez-GFP (green), Myc-Su(dx) (red) and DAPI (blue). White arrowheads indicate the change of Pez-GFP. Scale bar, 50 μm. (c) Overexpressing Su(dx)C917A cannot downregulate Pez-GFP. Adult fly midguts expressingUAS-Myc-Su(dx)-C917AbyMyo1Ats-Gal4were immunostained using Pez-GFP (green), Myc-Su(dx)C917A (red) and DAPI (blue). Scale bar, 50 μm. (d) RNAi knockdown of Su(dx) upregulates Pez-GFP. Adult fly midguts expressingUAS-Su(dx)-RNAibyMyo1Ats–Gal4was immunostained using Pez-GFP (green) and DAPI (blue). Scale bar, 50 μm. (e) Western blot analysis of samples in (a–d).Myo1Ats>Myc-Su(dx)decreased Pez-GFP protein levels whileMyo1Ats>Myc-Su(dx)C917Adid not affect Pez-GFP.Myo1Ats>Su(dx)RNAiinduced increase of Pez-GFP level. (f) Overexpression of Su(dx) inducesDrosophilaadult gut epithelial overgrowth. Guts from flies ofMyo1Ats-Gal4,Myo1Ats-Myc-Su(dx),Myo1Ats-Myc-Su(dx)C917Awere immnunostained to show actin (Phalloidin, red) and DAPI (blue). Scale bar, 50 μm. (g) Overexpression of Su(dx) induces increase of pH3-positive cell numbers inDrosophilaadult midgut. Guts from flies ofMyo1Ats,Myo1Ats-Myc-Su(dx),Myo1Ats-Myc-Su(dx)C917Awere immunostained by (PH3, red) and DAPI (blue). White arrows indicate the pH3-positive cells. Scale bar, 50 μm. (h) Quantification of PH3-positive cells per midgut of the indicated flies (n>4). The two-tailed Student’st-test was used to analyse the statistical significance. All data were shown as mean± s.e.m. *P<0.1, **P<0.01. ***P<0.001. (i) Su(dx) overexpression induces increased mRNA levels ofupd3andvn. To detect the mRNA levels ofupd3andvn, a real-time PCR analysis was induced. Error bars represent s.d. (n=3). The two-tailed Student’st-test was used to analyse the statistical significance. ***P<0.001, NS, no significance, versus control groups. (j–l) An increase of EGFR pathway activity was monitored in guts expressing Su(dx). Guts from flies ofMyo1Ats-Gal4 (j),Myo1Ats-Myc-Su(dx)(k) andMyo1Ats-Myc-Su(dx)-C917A(l) were stained to show GFP (green), dpERK (red) and DAPI (blue). Scale bar, 50 μm. Figure 2: Su(dx) overexpression in enterocytes induces Drosophila adult gut proliferation. ( a ) Pez distributes evenly in Drosophila midgut. Adult fly midguts expressing the GFP-tagged Pez genomic rescue construct (Pez-GFP) were immunostained with GFP (green) and DAPI (blue). Pez distributes evenly in Drosophila midgut. Scale bar, 50 μm. ( b ) Overexpressing Su(dx) induces Pez-GFP downregulation. Adult fly midguts expressing UAS-Myc-Su(dx) by Myo1A ts –Gal4 were immunostained using Pez-GFP (green), Myc-Su(dx) (red) and DAPI (blue). White arrowheads indicate the change of Pez-GFP. Scale bar, 50 μm. ( c ) Overexpressing Su(dx)C917A cannot downregulate Pez-GFP. Adult fly midguts expressing UAS-Myc-Su(dx)-C917A by Myo1A ts -Gal4 were immunostained using Pez-GFP (green), Myc-Su(dx)C917A (red) and DAPI (blue). Scale bar, 50 μm. ( d ) RNAi knockdown of Su(dx) upregulates Pez-GFP. Adult fly midguts expressing UAS-Su(dx)-RNAi by Myo1A ts –Gal4 was immunostained using Pez-GFP (green) and DAPI (blue). Scale bar, 50 μm. ( e ) Western blot analysis of samples in ( a – d ). Myo1A ts >Myc-Su(dx) decreased Pez-GFP protein levels while Myo1A ts >Myc-Su(dx)C917A did not affect Pez-GFP. Myo1A ts >Su(dx)RNAi induced increase of Pez-GFP level. ( f ) Overexpression of Su(dx) induces Drosophila adult gut epithelial overgrowth. Guts from flies of Myo1A ts -Gal4 , Myo1A ts -Myc-Su(dx) , Myo1A ts -Myc-Su(dx)C917A were immnunostained to show actin (Phalloidin, red) and DAPI (blue). Scale bar, 50 μm. ( g ) Overexpression of Su(dx) induces increase of pH3-positive cell numbers in Drosophila adult midgut. Guts from flies of Myo1A ts , Myo1A ts -Myc-Su(dx) , Myo1A ts -Myc-Su(dx)C917A were immunostained by (PH3, red) and DAPI (blue). White arrows indicate the pH3-positive cells. Scale bar, 50 μm. ( h ) Quantification of PH3-positive cells per midgut of the indicated flies ( n >4). The two-tailed Student’s t -test was used to analyse the statistical significance. All data were shown as mean± s.e.m. * P <0.1, ** P <0.01. *** P <0.001. ( i ) Su(dx) overexpression induces increased mRNA levels of upd3 and vn . To detect the mRNA levels of upd3 and vn , a real-time PCR analysis was induced. Error bars represent s.d. ( n =3). The two-tailed Student’s t -test was used to analyse the statistical significance. *** P <0.001, NS, no significance, versus control groups. ( j – l ) An increase of EGFR pathway activity was monitored in guts expressing Su(dx). Guts from flies of Myo1A ts -Gal4 ( j ), Myo1A ts -Myc-Su(dx) ( k ) and Myo1A ts -Myc-Su(dx)-C917A ( l ) were stained to show GFP (green), dpERK (red) and DAPI (blue). Scale bar, 50 μm. Full size image Previous studies have shown that loss of Pez induces intestinal hyperplasia and augments the activities of JAK/STAT and EGFR pathways [16] . We therefore speculated that overexpression of Su(dx) might produce similar phenotypes as when Pez is absent. Consistent with previous findings, Pez loss-of-function ( Pez 1/2 ) induced a hyperplasia of Drosophila midgut epithelium with an increase of Phospho-Histone3 (PH3)-positive cells and an elevation of unpaired3 (upd3) and vein (vn) transcription levels ( Supplementary Fig. 2b-d ). Overexpression of Su(dx), but not its C917A mutant, in EC cells using a Myo1A ts -Gal4 driver induced an obvious hyperplasia ( Fig. 2f ) with a marked increase of PH3-positive cells ( Fig. 2g,h ). Concomitantly, the transcription levels of upd3 and vn that represent JAK/STAT and EGFR activation were also significantly increased ( Fig. 2i ). Of note, upd3 expression was approximately 12-fold higher, whereas vn expression increased about twofold, compared with control guts ( Fig. 2i ). Furthermore, the elevation of EGFR pathway activity was reflected by the increase of dpERK level in midguts ( Fig. 2j–l ), which is similar to Pez loss-of-function phenotype ( Supplementary Fig. 2e,f ). These findings confirmed that Su(dx) overexpression induces similar overgrowth phenotypes as Pez loss-of-function does in midguts. In addition, we expressed Su(dx) and its C917A mutant in midgut ISCs and EBs using an escargot-Gal4 temperature-sensitive driver ( Esg ts ). Consistently, expression of Su(dx), but not Su(dx)C917A, slightly increased the numbers of PH3-positive cells and upregulated the activities of JAK/STAT and EGFR pathways ( Supplementary Fig. 2g–k ). Collectively, our results suggest that Su(dx) overexpression induces the proliferation of intestine resembling the phenotypes caused by the absence of Pez, and Su(dx) promotes Pez degradation to inhibit the function of Pez in midgut. Previous studies reported that Pez loss-of-function induces the proliferation of adult midgut ISCs yet does not affect intestinal cell differentiation ( Supplementary Fig. 3a–c ) [16] . On cell division, ISCs undergo self-renewal or proliferation to become enteroblasts (EBs), quiescent progenitor cells that ultimately differentiate into enterocytes (ECs) or enteroendocrine (ee) cells [13] , [22] . We then checked whether overexpressing Su(dx) in ECs affects cell differentiation in Drosophila midgut. According to the expression of EC marker Myo1A-GFP and ee cell marker Prospero (Pros), the numbers of ECs and ee cells were increased when Su(dx) was overexpressed in ECs. Overexpressed Su(dx) also induced increase of ISCs and EBs ( Supplementary Fig. 3d,e ). Also, the ratio of numbers of different cell types was not affected ( Supplementary Fig. 3g ). On the contrary, overexpression of Su(dx)C917A did not affect the numbers of ISCs, ECs or ee cells ( Supplementary Fig. 3f,g ). On the basis of these findings, we concluded that overexpression of Su(dx) promotes midgut cell proliferation but does not affect midgut cell differentiation. PY/ PPxY motifs and WW domains mediate Pez degradation To further explore the physical and functional interaction of Su(dx) and Pez, we first checked whether Pez and Su(dx) interact with each other by co-immunoprecipitation (Co-IP) assay in S2 cells. As shown in Fig. 3a , reciprocal interaction between Flag-Pez and Myc-Su(dx) was detected. We also found that overexpressed Myc-Su(dx) associated with endogenous Pez in S2 cells ( Supplementary Fig. 4a ). We then checked the localization of Pez and Su(dx) in S2 cells. When expressed alone in S2 cells, Flag-Pez was distributed evenly in the cytoplasm. Coexpression of Myc-Su(dx) changed the distribution pattern of Flag-Pez, and Myc-Su(dx) and Flag-Pez partially co-localized in cytoplasm ( Supplementary Fig. 4b–d ). 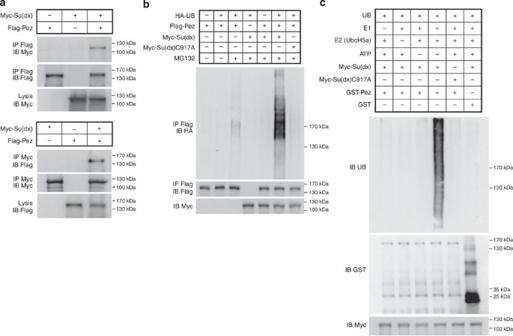Figure 3: Su(dx) ubiquitylates Pez bothin vivoandin vitro. (a) Pez binds with Su(dx) reciprocally in S2 cells. S2 cells were transfected with indicated constructs. Cell lysates were analysed by western blot analysis. (b) Su(dx) overexpression induces Pez ubiquitylation. S2 cells were co-transfected with indicated constructs. Cells were treated with MG132 (10 μm) for 4 h before harvesting. Immunoprecipitation was carried out with an anti-Flag antibody and followed by western blot analysis. (c) Su(dx) ubiquitylates Pezin vitro. Purified GST-Pez was incubated with Myc-Su(dx) or Myc-Su(dx)C917A (immuno-purified from transfected S2 cells), ubiquitin and E1, E2 (UbcH5a). After the reaction, the mixture was denatured and analysed by western blot. Figure 3: Su(dx) ubiquitylates Pez both in vivo and in vitro . ( a ) Pez binds with Su(dx) reciprocally in S2 cells. S2 cells were transfected with indicated constructs. Cell lysates were analysed by western blot analysis. ( b ) Su(dx) overexpression induces Pez ubiquitylation. S2 cells were co-transfected with indicated constructs. Cells were treated with MG132 (10 μm) for 4 h before harvesting. Immunoprecipitation was carried out with an anti-Flag antibody and followed by western blot analysis. ( c ) Su(dx) ubiquitylates Pez in vitro . Purified GST-Pez was incubated with Myc-Su(dx) or Myc-Su(dx)C917A (immuno-purified from transfected S2 cells), ubiquitin and E1, E2 (UbcH5a). After the reaction, the mixture was denatured and analysed by western blot. Full size image Because Su(dx) promotes Pez degradation in a proteasome-dependent manner ( Fig. 1b ), we tested whether Su(dx) mediates the ubiquitylation of Pez. As shown in Fig. 3b , Su(dx) markedly enhanced Pez ubiquitylation in a catalytic activity-dependent manner in S2 cells, which consists with the result of in vitro ubiquitylation experiment ( Fig. 3c ). It indicates that Su(dx) regulates Pez stability by promoting its ubiquitin-dependent proteomic degradation. Pez has a conserved PY motif (437aa–445aa: PTYRPAPDY, PY), a PPxY motif (553aa–556aa: PPPY) and a PPxxY motif (686aa–690aa: PPSGY), whereas Su(dx) contains four WW domains ( Fig. 4a ). It is well known that WW domains and proline-rich motifs mediate various protein–protein interactions [23] . To dissect whether proline-rich motifs and WW domains play a role in Pez degradation and Pez-Su(dx) interaction, several Su(dx) mutants and Pez mutants were constructed ( Fig. 4a and Supplementary Fig. 4e ). We cotransfected Su(dx) and different Pez mutants in S2 cells to check which Pez mutant can be stabilized. Finally, we found Pez-PA-PPPA mutant failed to be degraded by Su(dx) ( Fig. 4b and Supplementary Fig. 4f ). Furthermore, we noticed that Pez cannot be degraded by a Su(dx) truncation without WW domains (Su(dx)ΔWW) in S2 cells ( Fig. 4c ). In contrast, WW domains of Su(dx) exhibit a significant dominant negative activity and its co-expression stabilized Pez markedly ( Fig. 4d ). By co-immunoprecipitation experiments, we showed that Su(dx) WW domains are essential for Pez-Su(dx) association, as Su(dx)ΔWW does not interact with Pez ( Fig. 4e ). To minimize the interference of Su(dx)-induced degradation on detecting Pez-Su(dx) association, we used Su(dx) C917A mutant for the co-IP experiment to check the function of PY motif and PPPY motif of Pez. We found that PA and PPPA mutants markedly decreased the binding between Pez and Su(dx)C917A ( Fig. 4f ). Taken these results together, Su(dx)-induced Pez degradation depends on their physical interaction via WW domains and PY/PPPY motifs. This conclusion is also supported by the fact that Pez mutant containing PA and PPPA mutations cannot be ubiquitylated by Su(dx), compared with the wild-type Pez in S2 cells ( Fig. 4g ). To sum up, the binding of Pez to Su(dx) depends on PY/PPPY motifs of Pez and the WW domains of Su(dx), and is required for Su(dx)-mediated Pez degradation. 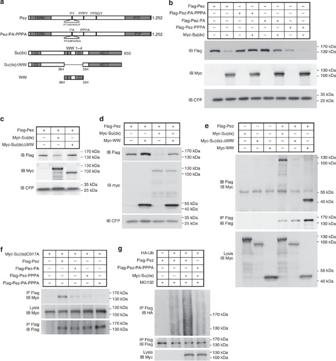Figure 4: Domains and motifs mediating the interaction between Su(dx) and Pez. (a) A schematic representation of Pez mutants and Su(dx) truncations. Pez contains an N-terminal FERM domain, a C-terminal PTP domain, a PPxY motif (PPPY), a PPxxY motif (PPSGY) and a proline-rich motif (PY). Su(dx) has an N-terminal C2 domain, a C-terminal HECT domain and four WW domains. (b) Pez-PA-PPPA mutant cannot be degraded by Su(dx). Flag-Pez mutants were transfected into S2 cells with or without Su(dx). Cell lysates were analysed using western blot. (c) Su(dx)ΔWW truncation cannot degrade Pez. Flag-Pez and Myc-Su(dx) or Myc-Su(dx)ΔWW were co-transfected into S2 cells. The cell lysates were analysed using western blot with the indicated antibodies. (d) Su(dx) WW domains stabilize Pez protein. Flag-Pez, Myc-WW and Myc-Su(dx) were co-transfected into S2 cells as indicated. Cell lysates were analysed using western blot. (e) WW domains of Su(dx) are required for its interaction with Pez. S2 cells were transfected with the indicated constructs. Immunoprecipitation was carried out with an anti-Flag antibody and followed by western blot analysis. (f) Pez PY and PPPY motifs are required for its interaction with Su(dx). S2 cells were transfected with the indicated constructs. Immunoprecipitation was carried out with an anti-Flag antibody followed by western blot analysis. (g) Pez PY and PPPY motifs are required for Pez ubiquitylation induced by Su(dx). S2 cells were transfected with the indicated constructs and treated with MG132 (10 μM) for 4 h before collection. Immunoprecipitation was carried out with an anti-Flag antibody followed by western blot analysis. Figure 4: Domains and motifs mediating the interaction between Su(dx) and Pez. ( a ) A schematic representation of Pez mutants and Su(dx) truncations. Pez contains an N-terminal FERM domain, a C-terminal PTP domain, a PPxY motif (PPPY), a PPxxY motif (PPSGY) and a proline-rich motif (PY). Su(dx) has an N-terminal C2 domain, a C-terminal HECT domain and four WW domains. ( b ) Pez-PA-PPPA mutant cannot be degraded by Su(dx). Flag-Pez mutants were transfected into S2 cells with or without Su(dx). Cell lysates were analysed using western blot. ( c ) Su(dx)ΔWW truncation cannot degrade Pez. Flag-Pez and Myc-Su(dx) or Myc-Su(dx)ΔWW were co-transfected into S2 cells. The cell lysates were analysed using western blot with the indicated antibodies. ( d ) Su(dx) WW domains stabilize Pez protein. Flag-Pez, Myc-WW and Myc-Su(dx) were co-transfected into S2 cells as indicated. Cell lysates were analysed using western blot. ( e ) WW domains of Su(dx) are required for its interaction with Pez. S2 cells were transfected with the indicated constructs. Immunoprecipitation was carried out with an anti-Flag antibody and followed by western blot analysis. ( f ) Pez PY and PPPY motifs are required for its interaction with Su(dx). S2 cells were transfected with the indicated constructs. Immunoprecipitation was carried out with an anti-Flag antibody followed by western blot analysis. ( g ) Pez PY and PPPY motifs are required for Pez ubiquitylation induced by Su(dx). S2 cells were transfected with the indicated constructs and treated with MG132 (10 μM) for 4 h before collection. Immunoprecipitation was carried out with an anti-Flag antibody followed by western blot analysis. Full size image To verify Pez–Su(dx) interaction in vivo , Flag-Pez or Flag-Pez-PA-PPPA was expressed either alone or together with Myc-Su(dx) in wing discs using a hh-Gal4 driver. Flag-Pez protein levels were decreased when coexpressed with Myc-Su(dx) while Flag-Pez-PA-PPPA protein levels were not affected ( Supplementary Fig. 5a–d ). We also checked the effect of Myc-Su(dx)ΔWW on Pez-GFP in wing discs. Overexpression of Myc-Su(dx)ΔWW by Ptc-Gal4 in wing discs did not affect Pez-GFP protein levels ( Supplementary Fig. 5e ). Furthermore, we used Myo1A ts -Gal4 to express Myc-Su(dx) with Pez or Pez-PA-PPPA. Coexpression with Pez or Pez-PA-PPPA rescued the excess number of pH3-positive cells and the increase of the mRNA level of Upd3/Vn induced by Myo1A ts -Su(dx) ( Supplementary Fig. 5f,g ). It is also worth noting that Pez-PA-PPPA had stronger function than Pez. Taken together, these observations suggest that the interaction between Pez and Su(dx) exists in vivo . Kibra inhibits Su(dx)-induced degradation to stabilize Pez We have demonstrated that WW domains of Su(dx) are required for its function in Pez degradation and its overexpression inhibited Su(dx) activity by a dominant-negative mechanism ( Fig. 4c,d ). Meanwhile, we noticed that Kibra, a reported Pez associated protein, also contains WW domains. Previous study showed that Kibra binds to Pez and co-localizes with Pez [16] . However, the function of Kibra in the Kibra–Pez complex is unclear. In our experiments, we found that Pez protein was significantly increased when Kibra is co-expressed in S2 cells ( Fig. 5a ). In contrast, Pez protein levels did not increase when co-expressed with a Kibra truncation that lacks WW domains (KibraΔWW), indicating that Kibra WW domains play an important role in regulating Pez stabilization. Furthermore, Kibra blocked Pez degradation induced by Su(dx) in a WW domain-dependent manner ( Fig. 5a ). Consistent with an earlier study, Kibra interacts with Pez in a WW domain-dependent manner ( Supplementary Fig. 6a ) [16] . Notably, we found PY and PPPY motifs were essential for the interaction between Kibra and Pez, as supported by the fact that Pez-PA-PPPA mutant was unable to bind to Kibra in vitro ( Supplementary Fig. 6b,c ). Accordingly, Pez-PA-PPPA mutant disrupted the co-localization between Kibra and Pez in S2 cells ( Supplementary Fig. 6d,e ). In addition, we knocked down Kibra in S2 cells using dsRNA to monitor the half-life of Pez. As shown in Fig. 5b,c , knockdown of Kibra accelerated the Pez turnover rate. The efficiency of Kibra knockdown is verified by a real-time PCR analysis ( Supplementary Fig. 6f ). Taken together, Kibra and Su(dx) antagonize each other to regulate Pez stability ( Fig. 5d ). Interestingly, neither Kibra nor Kibra-WW decreased the binding between Su(dx) and Pez ( Supplementary Fig. 6g ), suggesting Kibra may not function through competing with Su(dx) for Pez binding. 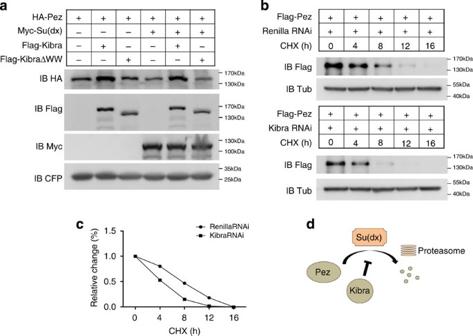Figure 5: Kibra stabilizes Pez in S2 cells and requires WW domains to exert this function. (a) Overexpressing Kibra stabilizes Pez in S2 cells. S2 cells were transfected with indicated constructs and cell lysates were analysed using western blot. Note that Pez was stabilized by Kibra but not Kibra-ΔWW. (b) Pez turnover rate is decreased after Kibra knockdown. S2 cells were transfected with Flag-Pez and treated with Renilla dsRNA or Kibra dsRNA. Cycloheximide (CHX, 100 μg ml−1) was added and cells were harvested at the indicated time points. Cell lysates were analysed using western blot. (c) Quantitative analysis of panels inb. (d) A model of the regulation of Pez protein stability by Su(dx) and Kibra. Su(dx) ubiquitylates and degrades Pez and this process is inhibited by Kibra. Figure 5: Kibra stabilizes Pez in S2 cells and requires WW domains to exert this function. ( a ) Overexpressing Kibra stabilizes Pez in S2 cells. S2 cells were transfected with indicated constructs and cell lysates were analysed using western blot. Note that Pez was stabilized by Kibra but not Kibra-ΔWW. ( b ) Pez turnover rate is decreased after Kibra knockdown. S2 cells were transfected with Flag-Pez and treated with Renilla dsRNA or Kibra dsRNA. Cycloheximide (CHX, 100 μg ml −1 ) was added and cells were harvested at the indicated time points. Cell lysates were analysed using western blot. ( c ) Quantitative analysis of panels in b . ( d ) A model of the regulation of Pez protein stability by Su(dx) and Kibra. Su(dx) ubiquitylates and degrades Pez and this process is inhibited by Kibra. Full size image PTPN14 is degraded by overexpressed Su(dx) or WWP1 As Pez and Su(dx) have conserved homologues in mammals, we tested whether the relationship between Su(dx) and Pez is conserved in mammals. In 293T cells, we co-transfected Su(dx) with human PTPN14, the closest orthologue of Pez. We found that, expression of Su(dx), but not Su(dx)C917A, markedly decreased the protein levels of PTPN14 ( Fig. 6a ). Notably, PTPN14 and Su(dx) interacted with each other in 293T cells ( Fig. 6b ). To address whether Su(dx) homologues promote PTPN14 degradation, we co-transfected PTPN14-SFB (S-tag, Flag epitope tag, and streptavidin-binding peptide tag) with different Su(dx) homologues, WWP1, WWP2 and Itch. PTPN14 protein levels were decreased specifically when WWP1 was co-transfected ( Fig. 6c ). Meanwhile, the degradation of PTPN14 induced by WWP1 overexpression was partially rescued by MG132 treatment ( Supplementary Fig. 7 ). Furthermore, WWP1–PTPN14 interaction was detected in two directions while WWP2–PTPN14 association was much weaker in one direction ( Fig. 6d ). These data might explain why WWP1 but not WWP2 induces obvious degradation of PTPN14. To summarize, we found overexpressed Su(dx) or its mammalian homologue WWP1 can induce degradation of PTPN14. 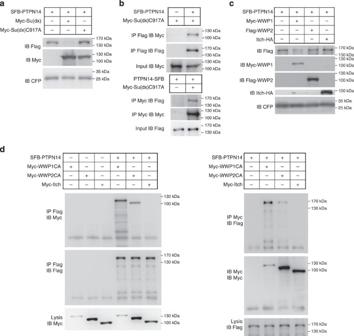Figure 6: PTPN14 is degraded by overexpressed Su(dx) or WWP1. (a) PTPN14, the human homologue of Pez, is degraded by Su(dx). The 293T cells were transfected with SFB-PTPN14 and Myc-Su(dx) or Myc-Su(dx)C917A. Cell lysates were analysed using western blot with the indicated antibodies. (b) PTPN14 interacts with Su(dx). The 293T cells were transfected with SFB-PTPN14 and Myc-Su(dx)C917A. Immunoprecipitation was carried out with the indicated antibodies and followed by western blot analysis. (c) PTPN14 protein levels are downregulated by WWP1. The 293T cells were transfected with the indicated constructs and cell lysates were analysed using western blot with the indicated antibodies. (d) PTPN14 binds to WWP1 or WWP2. The 293T cells were transfected with SFB-PTPN14 and Myc-WWP1CA, Myc-WWP2CA or Myc-Itch. Immunoprecipitation was carried out with the indicated antibodies and followed by western blot analysis. Figure 6: PTPN14 is degraded by overexpressed Su(dx) or WWP1. ( a ) PTPN14, the human homologue of Pez, is degraded by Su(dx). The 293T cells were transfected with SFB-PTPN14 and Myc-Su(dx) or Myc-Su(dx)C917A. Cell lysates were analysed using western blot with the indicated antibodies. ( b ) PTPN14 interacts with Su(dx). The 293T cells were transfected with SFB-PTPN14 and Myc-Su(dx)C917A. Immunoprecipitation was carried out with the indicated antibodies and followed by western blot analysis. ( c ) PTPN14 protein levels are downregulated by WWP1. The 293T cells were transfected with the indicated constructs and cell lysates were analysed using western blot with the indicated antibodies. ( d ) PTPN14 binds to WWP1 or WWP2. The 293T cells were transfected with SFB-PTPN14 and Myc-WWP1CA, Myc-WWP2CA or Myc-Itch. Immunoprecipitation was carried out with the indicated antibodies and followed by western blot analysis. Full size image Here we reported the identification of Su(dx) as an E3 ligase of Pez. Su(dx) was first identified as an E3 ligase regulating the Notch signalling pathway [17] , [18] , [24] , [25] . But the direct substrate of Su(dx) was unclear. In the present study, we identified Pez as a Su(dx) substrate. Furthermore, we checked whether Pez regulates the Notch signalling pathway. Pez knockdown induced notched wings and a decrease of Cut in wing discs that is very similar to what have caused by Su(dx) overexpression, indicating a dysfunction of the Notch pathway ( Supplementary Fig. 8a,b ). However, another typical marker of the Notch pathway, wingless, was not affected by the absence of Pez ( Supplementary Fig. 8c ). It is possible that Pez is not a canonical regulator of the Notch pathway and Su(dx) might have other substrates under this circumstance. According to our observations, Su(dx) overexpression in ECs only induced midgut epithelial proliferation to some extent, and it did not fully mimic the loss of pez induced phenotypes (compared Fig. 2f with Supplementary Fig. 2b ). We speculate that the difference was largely due to the incomplete degradation efficiency of Pez by Su(dx) overexpression in ECs. PTPN14 was reported as an inhibitor of YAP1 in mammalian cells. It can suppress the activity of YAP1 through retaining YAP1 in the cytoplasm and sustaining the phosphorylation state of YAP1 [8] . However, in our experiments, Pez overexpression slightly upregulates Yki phosphorylation level without obvious Yki localization change in S2 cells ( Supplementary Fig. 8d,e ). We speculated that the mechanism of YAP regulation by PTPN14 may not be conserved in Drosophila . Furthermore, our work present evidence that Kibra, a WW domain containing Pez partner, stabilizes Pez, providing an interesting model that WW–PY/PPxY interaction play a role in the regulation of protein stabilization ( Fig. 5d ). In addition, we found that other WW-containing proteins, such as Sav, were unable to stabilize Pez ( Supplementary Fig. 8f ). On the basis of these observations, we speculate the regulation of Pez stabilization by Su(dx) and Kibra is a specific event. We also found that PTPN14, the human homologue of Pez, can be degraded by overexpressed Su(dx) and its human homologue WWP1. However, in the following experiments, we found WWC1, the human homologue of Kibra, did not stabilize PTPN14 ( Supplementary Fig. 8g ). These data suggest that, although the similar regulation of Pez/PTPN14 by degradation exists in Drosophila and mammalian cells, the detailed mechanism may vary. It has been reported that PTPN14 sporadic mutations were found in breast cancer cells and colorectal cancer cells, indicating a potential tumour suppressor function of PTPN14. Moreover, amplification and overexpression of WWP1 has been found in breast and prostate cancers [26] , [27] , [28] , [29] . Therefore, our study may provide new insights into cancer development. Further characterization of the relationship of Su(dx)-Pez in mice and examination of their correlation in clinical cancers may provide potential targeting therapy for cancer treatments. Plasmids and cloning Pez full length was cloned from BDGP DGC clone. Mutation forms of Pez (Pez-PA, Pez-PPPA, Pez-PPSGA, Pez-PA-PPPA, Pez-PA-PPSGA, Pez-PPPA-PPSGA and Pez-PA-DA) were constructed according to the standard protocol. For expression in S2 cells and flies, constructs were cloned into the pUAST-Flag vector. To compare the activities of wild-type Pez and Pez-PA-PPPA, they were cloned into pUAST-attB vector for integrating into attP target site (75B) with ClonExpress II One Step Cloning Kit (Vazyme). PTPN14-SFB plasmid was a gift from Junjie Chen lab [8] . WWP1 and WWP2 cloned into pCDNA3.1 vector from human cDNA library. Itch-HA plasmid was provided by Lin Li lab [30] . All primers used in this study can be requested. Primers used for mutation constructs are as following: Pez-PPPA-F(5′- cccaccgccggccgtcaatcggc -3′); Pez-PPPA-R(5′- gccgattgacggccggcggtggg -3′); Pez-PPSGA-F(5′- gccgagtggagcccgtagttctg -3′); Pez-PPSGA-R(5′- cagaactacgggctccactcggc -3′); Pez-PA-F(5′- gctcgcccggcaccagacgctgagacggcggtc -3′); Pez-PA-R(5′- cagcgtctggtgccgggcgagctgtgggcagc -3′); Su(dx)-delWW-F(5′- cagcggatgatgagggtgctccgaaggg -3′); Su(dx)-delWW-R(5′- cccttcggagcaccctcatcatccgctg -3′). Drosophila genetics Fly stocks used in this study are as follows: Pez 1 , Pez 2 , Pez-GFP (gift from Hugo Stocker lab) [16] , Su(dx)-RNAi (gift from Dahua Chen lab) [31] , UAS-Myc-Su(dx) , UAS-Myc-Su(dx)C917A , UAS-Myc-Su(dx)ΔWW were generated according to standard P-element mediated transformation. Ptc-Gal4 , Hh-Gal4 , Diap3.5 (ref. 32 ), MyoAGal4; tubGal80ts , esgGal4; tubGal80ts [15] , Pez-RNAi (VDRC NO.30743), (Bloomington). All genetic experiments were conducted at 25 °C unless otherwise indicated. To induce conditional expression in adult flies, tub-Gal80ts flies were maintained at 18 °C though development, and then 2–6 day-old adult females were transferred to 29 °C for 7–9 days before dissection. Cell culture and transfection S2 cells were cultured in Schneider’s Medium (Invitrogen) with 10% heat-inactivated fetal bovine serum, 100 U ml −1 of penicillin and 100 mg ml −1 of Streptomycin at 25 °C. Transfection was carried out using Lipofectamine (Invitrogen) according to the manufacturer’s instructions. The cells were harvested 48 h after transfection. Ubiquitin-Gal4 construct was co-transfected with pUAST expression vectors in S2 cells. HEK293T cells were maintained at 37 °C in Dulbecco's Modified Eagle's Medium (DMEM) (Thermo) supplemented with 10% heat-inactivated fetal bovine serum and antibiotics with 5% CO 2 . For HEK293T cell transfection, Calcium Phosphate Transfection Kit (Specialty Media) was used according to the manufacturer’s instructions. Immunoprecipitation and immunostaining Immunoprecipitation was carried out at 4 °C. Cells were lysed in NP-40 buffer (50 mM pH8.0 Tris-HCl, 0.1 M NaCl, 10 mM NaF, 1 mM Na 3 VO 4 , 1% NP40, 10% Glycerol, 1.5 mM EDTA and Protease Inhibitor Cocktail). Lysates were first incubated with 2 μg indicated antibodies for 2 h and then with 20 μl protein A/G PLUS agaros (Santa Cruz Biotechnology) for 1 h. Beads were washed three times and boiled in SDS loading buffer. All raw western blot images are shown in Supplementary Fig. 9 . For cell immunostaining, cells were washed with PBS and fixed in 4% formaldehyde in PBS buffer at room temperature for 10 min, washed with PBS buffer and then treated with PBST (PBS and 0.25% Triton X-100) for permeabilization. Cells were blocked with PBSA (PBS and 1% BSA) for 15 min and then incubated with a primary antibody for 1 h in PBSA at room temperature, and then washed with PBS and incubated with a secondary antibody diluted in PBSA for 30 min at room temperature, and finally mounted in 40% glycerol. For imaginal disc staining and midgut staining, the third instar larvae or the adult flies from indicated genotypes were dissected. The samples were then fixed in 4% formaldehyde in PBS buffer, washed three times with PBS and incubated with primary and secondary antibodies in PBTA (PBS, 0.1% Triton X-100, and 1% BSA) buffer. 40% glycerol was used to mount the samples. Images of cells, imaginal discs and guts were acquired with a confocal microscope (LAS SP5; Leica) using a 40 × /1.25 NA oil objective (Leica) or 63 × /1.4 NA oil objective (Leica) at room temperature. To reduce the variables in experiments involving comparison between different genotypes, all samples were stained, processed and imagined in parallel. Images were then processed, scaled and analysed using Adobe Photoshop (Adobe). Antibodies used in this paper were as follows: mouse anti-Flag antibody (Sigma), mouse anti-Myc antibody (Santa Cruz), mouse anti-HA antibody (Sigma), mouse anti-GFP/CFP antibody (Santa Cruz), rabbit anti Pez antibody (generated by ABclonal Technology against Pez-C), Rat anti-Cubitus interruptus (Ci) antibody (Developmental Studies Hybridoma Bank, DSHB), Rabbit anti-lacZ antibody (Invitrogen), mouse anti Cut antibody (DSHB), rabbit anti-PH3 (1:300; Cell Signaling), mouse anti-Pros (1:20; DSHB), rabbit anti-dpERK (1:50; Cell Signaling) and rabbit anti-GFP (1:300; Invitrogen). RNA interference in Drosophila S2 Cells For RNAi in S2 cells, primers were designed as follows: kibra-dsRNA-F (5′- gaattaatacgactcactatagggagaagcgactgctttgggc -3′); kibra-dsRNA-R (5′- gaattaatacgactcactatagggagacaccgcaaagggatcg -3′);pez-dsRNA-1-F (5′- gaattaatacgactcactatagggagaactatctgaagaag -3′); pez-dsRNA-1-R (5′- gaattaatacgactcactatagggagaatgcgcagtcatatg -3′); pez-dsRNA-2-F (5′- gaattaatacgactcactatagggagacgccacgacaacatc -3′); pez-dsRNA-2-R (5′- gaattaatacgactcactatagggagagtagatgccaatcg -3′); Su(dx)-dsRNA-F (5′- gatcactaatacgactcactatagggtacatcaccctcatgacg -3′); Su(dx)-dsRNA-R (5′- gatcactaatacgactcactatagggtcattcctggcagaagcc -3′) PCR reactions were used as templates for in vitro RNA production ( in vitro Transcription T7 kit, Takara), and the RNA was purified using isopropyl-alcohol. dsRNA were then annealed (68 °C for 10 min and 37 °C for 30 min). To perform knockdown experiment, S2 cells were diluted into 1 × 10 6 cells ml −1 with serum-free medium for 1-h starvation with 15 μg ml −1 dsRNA. In vivo and in vitro ubiquitylation assay For in vivo ubiquitylation assay, S2 cells were transfected with indicated plasmids and treated with MG132 (100 μM ml −1 ) for 4 h before harvest. S2 cells were then lysed with 100 μl denaturing buffer (100 mM Tris-Cl pH 7.5, 10% SDS, 0.1 M DTT) and boiled for 10 min. The lysates were then diluted into 1 ml with NP40 buffer. Immunoprecipitation and western blot analysis were then carried out. For in vitro ubiquitylation assay, GST-Pez-loaded beads purified from E. coli were incubated with 100 ng E1 (Rabbit), 200 ng E2(UbcH5c), 5 mg ubiquitin (Boston Biochem), 2 mM ATP, and E3 in 20 μl ubiquitlyation buffer (50 mM Tris-Cl pH 7.5, 5 mM magnesium chloride, 2 mM sodium fluoride, 0.6 mM DTT, 10 nM Okadaic acid) at 30°C for 2 h. E3 (Myc-Su(dx) and Myc-Su(dx)C917A) were immunoprecipitated from transfected S2 cells and eluted by Myc peptides (Sigma). Real-time PCR RNA was isolated from S2 cells or female midguts at age 7–9 day-old. Coding DNA was synthesized with cDNA synthesis kit (Invitrogen). RT-PCR was performed on ABI Fast 7,500 using SYBR Green (Takara). Rp49 was used as normalization control. Primers for real-time PCR are as following: Su(dx)-qPCR-F (5′- attatggtggtgtatctc -3′); Su(dx)-qPCR-R (5′- ctgtagttgttcttgttc -3′); kibra-qPCR-F (5′- atcatcatcatcatcaac -3′); kibra-qPCR-R (5′- atctatgtaataggtcttg -3′); pez-qPCR-F (5′- gctaaccgaggatatgag -3′); pez-qPCR-R (5′- cctgatacacttggaact -3′); Vn-F (5′- tcacacatttagtggtggaagc -3′); Vn-R (5′- cgtgacctctgcgttctgt -3′); Upd3-F (5′- aaattcgacaaagtcgcctg -3′); Upd3-R (5′- ttccactggattcctggttc -3′); rp49-F (5′- cggatcgatatgctaagctgt -3′); rp49-R (5′- cgacgcactctgttgtcg -3′). Statistical analysis All statistical data were analysed using Student's t -test by R 2.9.0 and expressed as mean±s.e.m. Results were considered statistically significant when P <0.05. How to cite this article: Wang, C. et al . Suppressor of Deltex mediates Pez degradation and modulates Drosophila midgut homeostasis. Nat. Commun. 6:6607 doi: 10.1038/ncomms7607 (2015).